Methionine restriction extends lifespan ofDrosophila melanogasterunder conditions of low amino-acid status Reduced methionine (Met) intake can extend lifespan of rodents; however, whether this regimen represents a general strategy for regulating aging has been controversial. Here we report that Met restriction extends lifespan in both fruit flies and yeast, and that this effect requires low amino-acid status. Met restriction in Drosophila mimicks the effect of dietary restriction and is associated with decreased reproduction. However, under conditions of high amino-acid status, Met restriction is ineffective and the trade-off between longevity and reproduction is not observed. Overexpression of InRDN or Tsc2 inhibits lifespan extension by Met restriction, suggesting the role of TOR signalling in the Met control of longevity. Overall, this study defines the specific roles of Met and amino-acid imbalance in aging and suggests that Met restiction is a general strategy for lifespan extension. Calorie restriction (CR) as a means of extending lifespan has been used extensively in a variety of model organisms, such as yeast, nematodes, fruit flies, rats and mice [1] , [2] , [3] , [4] , [5] . Although the underlying mechanisms are not well understood, previous studies revealed the role of nutrient-sensing acting through TOR, which regulates metabolic processes and affects the rate of aging [6] , [7] , [8] , [9] . In spite of numerous studies involving CR, the dietary components responsible for this effect remain poorly characterized in most model systems. In fruit flies, restriction in dietary yeast extended lifespan, whereas a decrease in dietary sugar was ineffective, suggesting that specific component(s) of yeast include factor(s) that mediate the effect of dietary restriction [10] , [11] , [12] . It was also reported that methionine (Met) restriction mimics lifespan extension by CR in mice, providing one of the first examples of how a specific dietary factor could function to extend lifespan [13] , [14] , [15] , [16] , [17] . In previous studies involving CR and protein restriction in fruit flies, either dietary sugar and yeast dilution, or only dilution of dietary yeast, were used. Although these regimens were useful in addressing several critical questions, the identification of nutritional factors involved was not possible because one cannot remove a component from dietary yeast without changing other components [10] . To identify the specific nutrient factors that modulate longevity, several studies used semidefined or fully defined diets. For example, the use of a semidefined diet containing sugar and casein substituting for dietary protein revealed that the restriction in casein mimicked amino-acid restriction, thereby maximizing lifespan of Canton-S flies [18] . A recent study developed a fully defined diet that could be used to address the role of Met and other compounds in lifespan in fruit flies [19] . However, the initial studies that used this diet found no changes in the mean and maximum lifespan of non-virgin females when Met was restricted. Nutrient imbalance, particularly amino-acid imbalance, also received attention with regard to its influence on physiological function and modulation of aging. It was reported that disproportionate levels of amino acids may be associated with the incidence of adverse effects in a rat model. In particular, Met was defined as the most toxic amino acid when used in excess [20] . Restricted use of amino acids was suggested to be responsible for the lifespan extension caused by protein restriction [18] ; on the other hand, Met restriction was reported to be ineffective in extending lifespan of Drosophila [19] , [21] . Nevertheless, the roles of Met and its imbalance in aging remain largely uncharacterized, although potentially promising as lifespan extension by Met restriction was demonstrated in both rats and mice. If this effect is conserved across metazoa and beyond, other organisms including a commonly used model organism of aging, fruit flies, should also be subjected to lifespan extension by Met restriction. The use of defined diets varying in amino acids may provide an experimental system to examine the consequences of amino-acid imbalance and its effect on aging and other physiological functions. The role of Met in aging was also examined in studies that linked reproduction and longevity. It was reported that amino-acid imbalance caused by changes in Met levels differentially affected reproduction and longevity in Drosophila . This finding argued against the trade-off theory, wherein reproduction is inversely proportional to longevity [21] . It was unclear, however, how general this finding is, as only some conditions were examined. In the present study, we used the fully defined diet to characterize the parameters of aging and reproduction in fruit flies and yeast using Met diets varying in the levels of other amino acids. We describe the relationship between dietary Met, egg production and lifespan, and explain how Met status has an impact on lifespan depending on the status of other amino acids and acting through TOR signalling, establishing critical and specific roles of Met in aging. Sex-specific regulation of lifespan by high Met diet High Met intake is known to be toxic, presenting adverse effects on feeding, growth, pregnancy rate and sulfur metabolism in animals [22] , [23] , [24] , [25] , [26] . Thus, it is important to define the toxic range of dietary Met before its use in lifespan studies. In our study, we adopted a fully defined diet [19] , so that the levels of Met and its interaction with other amino acids and dietary components could be thoroughly examined. The 1.0X diet corresponding to 15% dietary yeast was supplemented with various amounts of Met and was used to analyse lifespan and egg production in Canton-S flies ( Fig. 1 and Supplementary Tables 1 and 2 ). Reduction of Met from 100 to 10 mM increased both the mean lifespan (21.65%, P< 0.0001, log-rank test) and reproduction (25.00%, P =0.039, Student’s t -test), suggesting that lifespan was increased by lowering Met toxicity. On the other hand, the reduction of Met from 10 to 1.5 mM did not affect lifespan ( P =0.9647, log-rank test) and decreased reproduction (−53.90%, P< 0.01, Student’s t -test), suggesting that Met toxicity was not involved at lower levels of this amino acid. 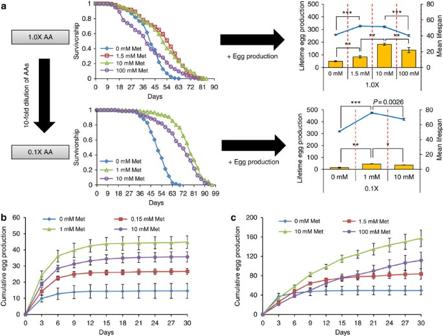Figure 1: Imbalance of amino acids and high levels of Met decrease lifespan and reproduction. (a) Survivorship curve, mean lifespan and lifetime egg production of mated female Canton-S flies reared on the 0.1X or 1.0X amino-acid diets containing 0, 1, 1.5, 10 or 100 mM Met were analysed. Bar graphs show lifetime egg production (left axis; mean±s.d.,n=40, *P<0.05, **P<0.01, Student’st-test) and line graphs mean lifespan (right axis; mean±s.e.m.,n=144~205, ***P<0.0001, log-rank test). SeeSupplementary Tables 1 and 2fornnumber and statistics of individual dietary groups. (b) Cumulative egg production of mated female Canton-S flies reared on the 0.1X diet containing 0, 0.15, 1 or 10 mM Met for 30 days (mean±s.d.,n=40). (c) Cumulative egg production of mated female Canton-S flies reared on the 1.0X diet containing 0, 1.5, 10 or 100 mM Met for 30 days (mean±s.d.,n=30). Figure 1: Imbalance of amino acids and high levels of Met decrease lifespan and reproduction. ( a ) Survivorship curve, mean lifespan and lifetime egg production of mated female Canton-S flies reared on the 0.1X or 1.0X amino-acid diets containing 0, 1, 1.5, 10 or 100 mM Met were analysed. Bar graphs show lifetime egg production (left axis; mean±s.d., n =40, * P< 0.05, ** P< 0.01, Student’s t -test) and line graphs mean lifespan (right axis; mean±s.e.m., n =144~205, *** P< 0.0001, log-rank test). See Supplementary Tables 1 and 2 for n number and statistics of individual dietary groups. ( b ) Cumulative egg production of mated female Canton-S flies reared on the 0.1X diet containing 0, 0.15, 1 or 10 mM Met for 30 days (mean±s.d., n =40). ( c ) Cumulative egg production of mated female Canton-S flies reared on the 1.0X diet containing 0, 1.5, 10 or 100 mM Met for 30 days (mean±s.d., n =30). Full size image To further define the Met toxicity range, we modified the original diet to reduce the levels of all amino acids tenfold (the 0.1X diet), varied Met (0, 1 and 10 mM) in this diet, and applied these dietary conditions to examine lifespan of Canton-S flies in conjunction with egg production ( Fig. 1 and Supplementary Tables 1 and 2 ). The mean lifespan was increased when Met was decreased from 10 to 1 mM (8.94%, P =0.0026, log-rank test), and this effect was accompanied by an increase in egg production (20.17%, P =0.048, Student’s t -test), suggesting that a decrease in Met toxicity contributes to an increase in lifespan here as well. To further examine the toxic effect of Met, the 0.1X diet containing 0.15, 1 or 10 mM Met was applied to analyse lifespan of Canton-S, Oregon-R and w 1118 flies under mixed-sex conditions ( Figs 2 and 3 and Supplementary Table 3 ). 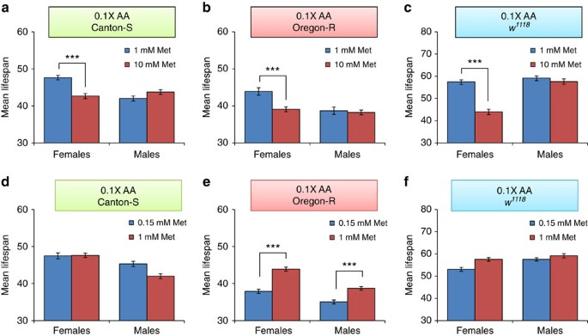Figure 3: Sex-specific decrease of lifespan by imbalance of amino acids and high levels of Met. (a–c) Female and male Canton-S, Oregon-R andw1118flies reared on the 0.1X diet containing 1 or 10 mM Met. (a) Canton-S (mean±s.e.m.,n=184~196), (b) Oregon-R (mean±s.e.m.,n=198~206) and (c)w1118(mean±s.e.m.,n=81~94) flies were analysed for the mean lifespan and examined for differences among dietary groups (***P<0.0001, log-rank test). (d–f) Female and male Canton-S, Oregon-R andw1118flies reared on the 0.1X diet containing 0.15 or 1 mM Met. (d) Canton-S (mean±s.e.m.,n=187~196), (e) Oregon-R (mean±s.e.m.,n=198~203) and (f)w1118(mean±s.e.m.,n=91~99) flies were analysed for the mean lifespan and analysed for differences among dietary groups (***P<0.0001, log-rank test). SeeSupplementary Table 3fornnumber and statistics of individual strains and dietary group. The mean lifespan of female flies increased when Met was reduced from 10 to 1 mM (Canton-S: 10.48%, P =0.0308; Oregon-R: 10.98%, P =0.0119: w 1118 : 23.60%, P< 0.0001, log-rank test), whereas no difference was observed in males (Canton-S: P =0.1239; Oregon-R: P =0.5754; w 1118 : P =0.8623, log-rank test). Furthermore, no effect on lifespan was seen in both male and female flies when Met was reduced from 1 to 0.15 mM. Thus, the 10 mM Met-0.1X diet was toxic to female flies only (it decreased both lifespan and reproduction). Our data suggested that the 1 mM Met-0.1X diet (a tenfold dilution from the original 10 mM-1X diet) was balanced. Interestingly, dietary Met toxicity was observed only in 100 mM Met-1X and 10 mM Met-0.1X diets that clearly represent Met imbalance (high Met levels when the levels of other amino acids are low). On the other hand, lifespan was not changed between the 10 mM Met-1X and 1.5 mM Met-1X diets. These findings show that the imbalance of Met relative to other amino acids (rather than the presence of high Met) is the reason for the reduction in both longevity and reproduction. 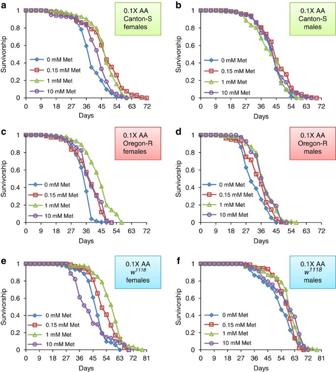These findings established the toxic range of Met and showed that its toxicity is limited to female flies and depends on its interaction with other amino acids. Figure 2: Survivorship curves of fruit flies reared on the 0.1X diet varying in Met levels. (a) Female Canton-S flies, (b) male Canton-S flies, (c) female Oregon-R flies, (d) male Oregon-R flies, (e) femalew1118flies and (f) malew1118flies were reared on the 0.1X diet containing 0, 0.15, 1 or 10 mM Met are shown in the survivorship curves. Figure 2: Survivorship curves of fruit flies reared on the 0.1X diet varying in Met levels. ( a ) Female Canton-S flies, ( b ) male Canton-S flies, ( c ) female Oregon-R flies, ( d ) male Oregon-R flies, ( e ) female w 1118 flies and ( f ) male w 1118 flies were reared on the 0.1X diet containing 0, 0.15, 1 or 10 mM Met are shown in the survivorship curves. Full size image Figure 3: Sex-specific decrease of lifespan by imbalance of amino acids and high levels of Met. ( a – c ) Female and male Canton-S, Oregon-R and w 1118 flies reared on the 0.1X diet containing 1 or 10 mM Met. ( a ) Canton-S (mean±s.e.m., n =184~196), ( b ) Oregon-R (mean±s.e.m., n =198~206) and ( c ) w 1118 (mean±s.e.m., n =81~94) flies were analysed for the mean lifespan and examined for differences among dietary groups (*** P< 0.0001, log-rank test). ( d – f ) Female and male Canton-S, Oregon-R and w 1118 flies reared on the 0.1X diet containing 0.15 or 1 mM Met. ( d ) Canton-S (mean±s.e.m., n =187~196), ( e ) Oregon-R (mean±s.e.m., n =198~203) and ( f ) w 1118 (mean±s.e.m., n =91~99) flies were analysed for the mean lifespan and analysed for differences among dietary groups (*** P< 0.0001, log-rank test). See Supplementary Table 3 for n number and statistics of individual strains and dietary group. Full size image Lifespan extension by Met and amino-acid restriction It was recently found that neither Met restriction nor Met excess affected the lifespan of mated female flies in the context of normal or CR diets [19] , [21] . In contrast, metformin-induced Met restriction extended the lifespan of nematodes [27] , and the lifespan could also be extended by Met restriction in mice and rats [14] , [15] , [16] . This discrepancy in the effect of Met restriction in model organisms raised questions regarding evolutionary conservation and general applicability of the Met restriction strategy. To examine this issue, we focused on the interaction of Met with other amino acids. This interaction brings complexity to lifespan studies, which has not been previously characterized—for example, Met restriction may reduce translation and reproduction thereby increasing lifespan, whereas it may also lead to an accumulation of unused amino acids thereby decreasing lifespan. To define the role of Met in aging as a function of amino-acid status, we employed diets with different levels of amino acids (0.4X corresponding to 6% dietary yeast, 0.7X corresponding to 10.5% dietary yeast and 1.0X corresponding to 15% dietary yeast) and different Met concentrations (0, 0.15 and 1 mM). We subjected mated Canton-S female flies to these diets and determined their lifespan and egg production ( Fig. 4 and Supplementary Tables 4–6 ). 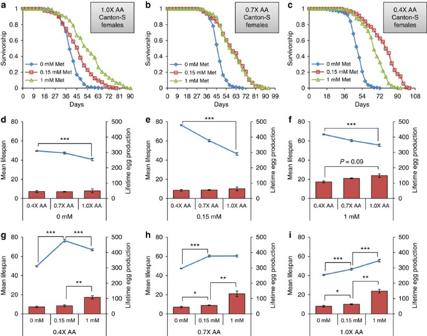Figure 4: Lifespan extension of mated female flies by Met restriction and low amino acids. (a–c) Survivorship curves of mated female Canton-S flies reared on (a) 1.0X diet containing 0, 0.15 or 1 mM Met, (b) 0.7X diet containing 0, 0.15 or 1 mM Met, or (c) 0.4X diet containing 0, 0.15 or 1 mM Met, are shown. The mean lifespan and lifetime egg production of mated female Canton-S flies on (d) 0.4X, 0.7X or 1.0X diets containing 0 mM Met (mean lifespan: mean±s.e.m.,n=134~151, ***P<0.0001, log-rank test; lifetime egg production: mean±s.d.,n=40, *P<0.05, **P<0.01, Student’st-test), (e) 0.4X, 0.7X or 1.0X diets containing 0.15 mM Met (mean lifespan: mean±s.e.m.,n=123~150, ***P<0.0001, log-rank test; lifetime egg production: mean±s.d.,n=40, *P<0.05, **P<0.01, Student’st-test), (f) 0.4X, 0.7X or 1.0X diets containing 1 mM Met (mean lifespan: mean±s.e.m.,n=144~150, ***P<0.0001, log-rank test; lifetime egg production: mean±s.d.,n=40, *P<0.05, **P<0.01, Student’st-test), (g) 0.4X diet containing 0, 0.15 or 1 mM Met (mean lifespan: mean±s.e.m.,n=123~150, ***P<0.0001, log-rank test; lifetime egg production: mean±s.d.,n=40, *P<0.05, **P<0.01, Student’st-test), (h) 0.7X diet containing 0, 0.15 or 1 mM Met (mean lifespan: mean±s.e.m.,n=150~151, ***P<0.0001, log-rank test; lifetime egg production: mean±s.d.,n=40, *P<0.05, **P<0.01, Student’st-test), (i) 1.0X diet containing 0, 0.15 or 1 mM Met (mean lifespan: mean±s.e.m.,n=134~144, ***P<0.0001, log-rank test; lifetime egg production: mean±s.d.,n=40, *P<0.05, **P<0.01, Student’st-test), are shown. Bar graphs show lifetime egg production (right axis) and line graphs mean lifespan (left axis). SeeSupplementary Tables 4–6fornnumber and statistics of individual dietary groups. Figure 4: Lifespan extension of mated female flies by Met restriction and low amino acids. ( a – c ) Survivorship curves of mated female Canton-S flies reared on ( a ) 1.0X diet containing 0, 0.15 or 1 mM Met, ( b ) 0.7X diet containing 0, 0.15 or 1 mM Met, or ( c ) 0.4X diet containing 0, 0.15 or 1 mM Met, are shown. The mean lifespan and lifetime egg production of mated female Canton-S flies on ( d ) 0.4X, 0.7X or 1.0X diets containing 0 mM Met (mean lifespan: mean±s.e.m., n =134~151, *** P< 0.0001, log-rank test; lifetime egg production: mean±s.d., n =40, * P< 0.05, ** P< 0.01, Student’s t -test), ( e ) 0.4X, 0.7X or 1.0X diets containing 0.15 mM Met (mean lifespan: mean±s.e.m., n =123~150, *** P< 0.0001, log-rank test; lifetime egg production: mean±s.d., n =40, * P< 0.05, ** P< 0.01, Student’s t -test), ( f ) 0.4X, 0.7X or 1.0X diets containing 1 mM Met (mean lifespan: mean±s.e.m., n =144~150, *** P< 0.0001, log-rank test; lifetime egg production: mean±s.d., n =40, * P< 0.05, ** P< 0.01, Student’s t -test), ( g ) 0.4X diet containing 0, 0.15 or 1 mM Met (mean lifespan: mean±s.e.m., n =123~150, *** P< 0.0001, log-rank test; lifetime egg production: mean±s.d., n =40, * P< 0.05, ** P< 0.01, Student’s t -test), ( h ) 0.7X diet containing 0, 0.15 or 1 mM Met (mean lifespan: mean±s.e.m., n =150~151, *** P< 0.0001, log-rank test; lifetime egg production: mean±s.d., n =40, * P< 0.05, ** P< 0.01, Student’s t -test), ( i ) 1.0X diet containing 0, 0.15 or 1 mM Met (mean lifespan: mean±s.e.m., n =134~144, *** P< 0.0001, log-rank test; lifetime egg production: mean±s.d., n =40, * P< 0.05, ** P< 0.01, Student’s t -test), are shown. Bar graphs show lifetime egg production (right axis) and line graphs mean lifespan (left axis). See Supplementary Tables 4–6 for n number and statistics of individual dietary groups. Full size image With regard to the role of amino-acid status, we found that lifespan could be extended by amino-acid restriction at any Met concentration ( Fig. 4a–f and Supplementary Tables 4–6 ). For example, when comparing 0.4X and 1.0X diets, the mean lifespan increased 22.09% at 0 mM Met ( P< 0.0001, log-rank test), 64.1% at 0.15 mM Met ( P< 0.0001, log-rank test) and 20.17% at 1 mM Met ( P< 0.0001, log-rank test). It was previously reported that a lower intake of casein that substitutes for dietary yeast protein increases fruit fly lifespan, suggesting that amino-acid restriction can extend lifespan and that this effect may possibly explain lifespan extension by dietary restriction [18] , [21] . Our findings also support the idea that amino-acid restriction could extend lifespan of mated female flies maintained on the fully defined diet. However, an amino-acid restriction that does not affect reproduction, body mass and total protein (for example, see the data for 0 mM Met in Figs 4 and 5 and Supplementary Tables 4–6 ) could still lead to lifespan extension. Although food consumption increased at low amino-acid levels, it could not contribute to the lifespan extension by amino-acid restriction due to its negative regulation of aging ( Fig. 5 ). Overall, amino-acid restriction extended lifespan at any Met level (including Met deficiency, when it did not affect reproduction). 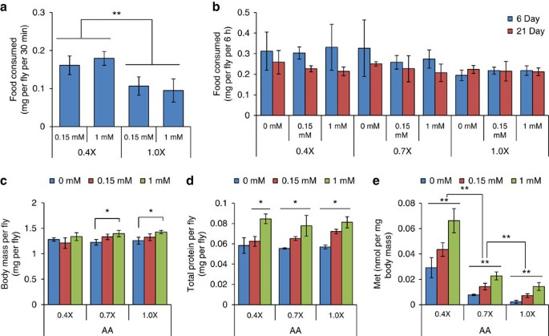Figure 5: Analysis of eating behaviour and endogenous Met concentration of mated female flies. (a–e) Flies were reared on 0.4X, 0.7X or 1.0X diets containing 0, 0.15 or 1 mM Met, and then collected on 6th or 21st days. (a) Food consumption for 30 min on the 6th day (mean±s.d.,n=100) and (b) food consumption for 6 h on the 6th and 21st days (mean±s.d.,n=20) were analysed via a feeding assay using erioglaucine. (c) Body mass (per fly) (mean±s.d.,n=75), (d) total protein (per fly; mean±s.d.,n=75), (e) amounts of endogenous Met normalized to body mass (mean±s.d.,n=75) were analysed on the 21st day. All experiments were repeated three to 10 times independently and statistics was assessed by using Student’st-test (*P<0.05 and **P<0.01). Figure 5: Analysis of eating behaviour and endogenous Met concentration of mated female flies. ( a – e ) Flies were reared on 0.4X, 0.7X or 1.0X diets containing 0, 0.15 or 1 mM Met, and then collected on 6th or 21st days. ( a ) Food consumption for 30 min on the 6th day (mean±s.d., n =100) and ( b ) food consumption for 6 h on the 6th and 21st days (mean±s.d., n =20) were analysed via a feeding assay using erioglaucine. ( c ) Body mass (per fly) (mean±s.d., n =75), ( d ) total protein (per fly; mean±s.d., n =75), ( e ) amounts of endogenous Met normalized to body mass (mean±s.d., n =75) were analysed on the 21st day. All experiments were repeated three to 10 times independently and statistics was assessed by using Student’s t -test (* P< 0.05 and ** P< 0.01). Full size image With regard to the effect of Met status, Met restriction extended lifespan depending on the status of other amino acids ( Fig. 4a–c, g–i and Supplementary Tables 4–6 ). For example, when comparing 1.0X and 0.7X diets, Met restriction decreased (or did not change) the mean lifespan, whereas on the 0.15 mM Met-0.4X diet the lifespan was 12.53% higher than on the 1 mM Met-0.4X diet ( P< 0.0001, log-rank test). Moreover, Met restriction was accompanied by decreased reproduction, suggesting that the observed lifespan extension was mechanistically different from the effect of decreased Met toxicity. We further analysed food consumption rate, determining whether Met status influenced eating behaviour that in turn affected lifespan ( Fig. 5 ). Interestingly, food consumption was not affected by dietary Met. Thus, lifespan can be extended in fruit flies by Met restriction, as it can in rodents, but this effect requires low amino-acid status. Interplay between lifespan and reproduction The cost-of-reproduction is an important factor that may affect lifespan as a part of evolutionary trade-offs involving maintenance and reproduction. However, it was reported that under CR conditions the addition of Met did not affect lifespan, yet increased reproduction, suggesting exception from the trade-off theory [21] . To understand this phenomenon, we quantified egg production by Canton-S flies and compared it with the mean lifespan of mated female flies in two ways: using three different levels of amino acids at a constant Met concentration ( Fig. 4d–f and Supplementary Tables 4–7 ); and using three Met concentrations at a constant amino-acid level ( Fig. 4g–i and Supplementary Tables 4–7 ). As expected, Met status could limit reproduction. In particular, there was no difference in reproduction between 0 mM Met-0.4X and 0 mM Met-1.0X diets ( P =0.828, Student’s t -test; Fig. 4d and Supplementary Tables 4–6 ). Moreover, an increase in Met levels correlated with an increase in lifetime egg production on each amino-acid diet ( Fig. 4g–i and Supplementary Tables 4–6 ). We also examined how Met status affected gene expression by generating microarray data for the examined conditions. Gene clustering following stringent filtering with permutation revealed that most genes downregulated by Met restriction in either 0.4X or 1.0X diets were linked to egg production ( Fig. 6 and Supplementary Data 1 ), whereas this was not the case under conditions of amino-acid restriction, even when less stringent filtering was applied ( Fig. 6b and Supplementary Data 1 ). These data suggest that Met plays a key regulatory role in reproduction, whereas the gene expression analyses suggested that the status of other amino acids was more relevant to regulation of functions, such as heme-binding, iron–ion binding, microsome, monooxygenase activity and oxidoreductase activity ( Fig. 6 ). On the other hand, the mean lifespan decreased with the increased supply of amino acids at any Met concentration, whereas reproduction was not changed with the increased supply of amino acids during Met deficiency ( Fig. 4d–f and Supplementary Tables 4–6 ). Thus, the data suggest that the change in reproduction may not underlie lifespan extension by amino-acid restriction, resulting in the appearance of exception from the trade-off under conditions of limited Met supply. 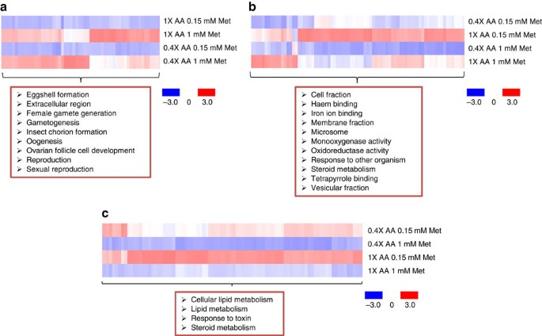Figure 6: Gene clusters whose expression is regulated by Met restriction and amino-acid levels. (a–c) Mated female Canton-S flies (n=30) were raised on the 0.4X amino-acid diet containing 0.15 or 1 mM Met, or the 1X amino-acid diet containing 0.15 or 1 mM Met for 18 days, and gene expression was examined by microarray analyses. (a) Gene clusters, whose expression was reduced by Met restriction in both amino-acid diets, and (b) decreased by low levels of amino acids in both Met diets are shown. (c) Gene clusters that were upregulated by Met restriction in both amino-acid diets are shown. Figure 6: Gene clusters whose expression is regulated by Met restriction and amino-acid levels. ( a – c ) Mated female Canton-S flies ( n =30) were raised on the 0.4X amino-acid diet containing 0.15 or 1 mM Met, or the 1X amino-acid diet containing 0.15 or 1 mM Met for 18 days, and gene expression was examined by microarray analyses. ( a ) Gene clusters, whose expression was reduced by Met restriction in both amino-acid diets, and ( b ) decreased by low levels of amino acids in both Met diets are shown. ( c ) Gene clusters that were upregulated by Met restriction in both amino-acid diets are shown. Full size image When comparing changes in lifespan and reproduction between 0.15 and 1 mM Met diets (and the same amino-acid status), the mean lifespan increased 12.53% on the 0.15 mM Met-0.4X diet ( P< 0.0001, log-rank test), decreased 19.44% on the 0.15 mM-1X diet ( P< 0.0001, log-rank test), and showed no difference on the 0.15 mM Met-0.7X diet ( P =0.9842, log-rank test), whereas reproduction decreased 103.8% on the 0.15 mM Met-0.4X diet, 135.45% on the 0.15 mM Met-0.7X diet and 135.38% on the 0.15 mM Met-1.0X diet ( P< 0.01, Student’s t -test) ( Fig. 4g–i and Supplementary Tables 4–7 ). 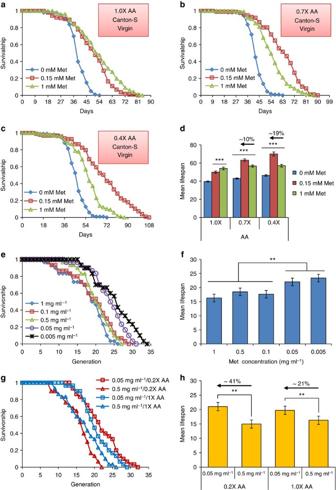Figure 7: Lifespan extension of virgin female flies and yeast by Met restriction. (a–c) Survivorship curves of virgin Canton-S flies reared on (a) 0.4X diet containing 0, 0.15 or 1 mM Met, (b) 0.7X diet containing 0, 0.15 or 1 mM Met or (c) 1.0X diet containing 0, 0.15 or 1 mM Met are shown. (d) The mean lifespan of virgin flies on these diets was compared (mean±s.e.m.,n=92~111, ***P<0.0001, log-rank test). SeeSupplementary Tables 8 and 9fornnumber and statistics of individual dietary groups. (e) Survivorship curves and (f) the mean lifespan of yeast grown on defined medium containing 1, 0.1, 0.5, 0.05 or 0.005 mg ml−1Met (mean±s.e.m.,n=30, **P<0.01, Rank-sum test). (g) Survivorship curve and (h) the mean lifespan of yeast grown on defined media containing 0.5 or 0.05 mg ml−1Met under conditions of 0.2X or 1.0X amino-acid status (mean±s.e.m.,n=30, **P<0.01, Rank-sum test). SeeSupplementary Tables 10 and 11for statistics of individual dietary groups. Accordingly, a decrease in reproduction due to Met deficiency did not coincide with the increase in lifespan under conditions of high amino-acid status (for example, 0.7X and 1.0X diets), whereas a decrease in reproduction due to Met deficiency inversely correlated with the lifespan increase on the low amino-acid status (for example, 0.4X diet; Pearson’s coefficient: −0.963~−0.864, P< 0.0021~0.0265; Supplementary Table 7 ). Thus, lifespan extension by Met restriction under conditions of low amino-acid status was accompanied by decreased reproduction, suggesting that the trade-off may be observed, at least under certain conditions. Lifespan extension by Met restriction in virgin flies We tested whether the observed lifespan extension of mated female flies by Met deficiency also applies to flies under other conditions. To examine these possibilities, virgin Canton-S flies were subjected to the same diets with varying Met and amino-acid levels ( Fig. 7a–d and Supplementary Tables 8 and 9 ). Indeed, the effects observed with mated female flies were reproduced with the virgin flies. The mean lifespan of virgin flies reared on the 0.15 mM Met-0.4X diet was ~19% higher than on the 1 mM Met-0.4X diet, and lifespan on the 0.15 mM Met-0.7X diet was ~10% higher than on the 1 mM Met-0.7X diet (0.15 mM Met- and 1 mM Met-0.4X; P< 0.0001, 0.15 mM Met- and 1 mM Met-1.0X; P =0.0001, log-rank test). On the other hand, Met reduction from 1 to 0.15 mM on the 1.0X diets did not increase lifespan (−8.31%, P =0.0085, log-rank test). These data support the finding that the lifespan extension by Met restriction is maximized at low levels of other amino acids. Figure 7: Lifespan extension of virgin female flies and yeast by Met restriction. ( a – c ) Survivorship curves of virgin Canton-S flies reared on ( a ) 0.4X diet containing 0, 0.15 or 1 mM Met, ( b ) 0.7X diet containing 0, 0.15 or 1 mM Met or ( c ) 1.0X diet containing 0, 0.15 or 1 mM Met are shown. ( d ) The mean lifespan of virgin flies on these diets was compared (mean±s.e.m., n =92~111, *** P< 0.0001, log-rank test). See Supplementary Tables 8 and 9 for n number and statistics of individual dietary groups. ( e ) Survivorship curves and ( f ) the mean lifespan of yeast grown on defined medium containing 1, 0.1, 0.5, 0.05 or 0.005 mg ml −1 Met (mean±s.e.m., n =30, ** P< 0.01, Rank-sum test). ( g ) Survivorship curve and ( h ) the mean lifespan of yeast grown on defined media containing 0.5 or 0.05 mg ml −1 Met under conditions of 0.2X or 1.0X amino-acid status (mean±s.e.m., n =30, ** P< 0.01, Rank-sum test). See Supplementary Tables 10 and 11 for statistics of individual dietary groups. Full size image Extension of yeast lifespan by Met restriction We also examined another common model organism of aging, the budding yeast. Yeast replicative lifespan was assayed in cells grown on the medium containing various Met levels (0.1, 0.5, 0.05, 0.005 or 1 mg ml −1 ) ( Fig. 7e–h and Supplementary Tables 10 and 11 ). Two lowest Met levels (0.05 and 0.005 mg ml −1 Met) were most effective in extending yeast lifespan, suggesting that the findings in fruit flies may apply to yeast. On the basis of these results, we further changed the amino-acid status for 0.5 and 0.05 mg ml −1 Met conditions and observed a significant increase (4.4 generations; P =0.004, rank-sum test) in the mean lifespan upon reducing Met. Met decrease was also effective in extending lifespan in other media (0.2X, 1X and 5X), but the low amino-acid status was the most effective. Thus, low amino-acid status maximizes the lifespan extension by Met restriction in yeast, suggesting both a general applicability of Met restriction in extending lifespan and the dependence of this effect on low amino-acid status. Lifespan control by Met restriction requires the TOR pathway It was reported that the effect of dietary restriction on lifespan was due to inhibition of TOR signalling [7] , [8] , [9] . We reasoned that the lifespan extension by Met restriction may also involve TOR inhibition. To test this possibility, we used two transgenic lines of fruit flies containing an upstream activating sequence linked to a dominant-negative form of Drosophila insulin receptor ( UAS-dInRDN ) or to Drosophila Tsc2 ( UAS-dTsc2 ). Mated female flies that overexpress either InRDN or Tsc2 were subjected to four diets (1 mM Met-1X, 0.2 mM Met-1X, 1 mM Met-0.4X, 0.2 mM Met-0.4X) and their lifespan was analysed ( Fig. 8 and Supplementary Tables 12 and 13 ). We found that the mean lifespan of control flies ( +/UAS-dInRDN and +/UAS-dTsc2 ) was differentially regulated by Met restriction upon changes in amino-acid status ( Fig. 8a–h and Supplementary Tables 12 and 13 ). For example, Met decrease from 1 to 0.2 mM in the 1.0X diet decreased lifespan in both control lines ( +/UAS-dInRDN , −12.82%, P< 0.0001; +/UAS-dTsc2 , −17.85%, P< 0.0001, log-rank test), whereas it extended lifespan when the flies were on the 0.4X diet ( +/UAS-dInRDN , 15.86%, P< 0.0001; +/UAS-dTsc2 , 4.03%, P =0.01, log-rank test). Interestingly, Met decrease from 1 to 0.2 mM on the 0.4X diet did not extend lifespan of da-Gal4 > UAS-dInRDN (−2.88%, P =0.10, log-rank test) and da-Gal4 > UAS-dTsc2 (−21.88%, P< 0.0001, log-rank test) lines ( Fig. 8e–h and Supplementary Tables 12 and 13 ). These data suggest that overexpression of InRDN or Tsc2, which inactivate TOR signalling, inhibited lifespan extension by Met restriction. Thus, similar to the CR case, the lifespan extension by Met restriction under conditions of low amino acids utilizes the inhibition of TOR signalling. 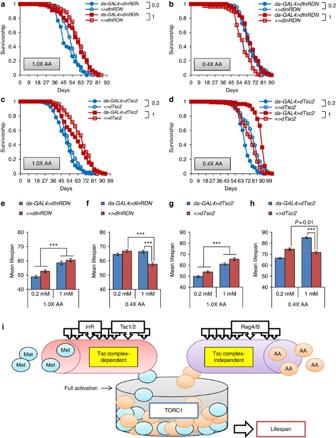Figure 8: Role of TOR signalling in lifespan extension by Met restriction. (a–d) Survivorship curves ofda-GAL4>dInRDNand+>dInRDNreared on (a) 1.0X diet containing 0.2 or 1 mM Met, (b) 0.4X diet containing 0.2 or 1 mM Met. Survivorship curves ofda-GAL4>dTsc2and+>dTsc2reared on (c) 1.0X diet containing 0.2 or 1 mM Met, (d) 0.4X diet containing 0.2 or 1 mM Met. 0.2 and 1 correspond to 0.2 mM Met and 1 mM Met, respectively. (e,f) The mean lifespan ofda-GAL4>dInRDNand+>dInRDNreared on (e) 1.0X diet containing 0.2 or 1 mM Met (mean±s.e.m.,n=81~106, ***P<0.0001, log-rank test), (f) 0.4X diet containing 0.2 or 1 mM Met (mean±s.e.m.,n=88~106, ***P<0.0001, log-rank test). (g,h) The mean lifespan ofda-GAL4>dTsc2and+>dTsc2reared on (g) 1.0X diet containing 0.2 or 1 mM Met (mean±s.e.m.,n=104~149, ***P<0.0001, log-rank test), (h) 0.4X diet containing 0.2 or 1 mM Met (mean±s.e.m.,n=111~152, ***P<0.0001, log-rank test). SeeSupplementary Tables 12 and 13fornnumber and statistics of individual strains and dietary groups. (i) Model of TORC1 activation by Met and amino acids. Figure 8: Role of TOR signalling in lifespan extension by Met restriction. ( a – d ) Survivorship curves of da-GAL4>dInRDN and +>dInRDN reared on ( a ) 1.0X diet containing 0.2 or 1 mM Met, ( b ) 0.4X diet containing 0.2 or 1 mM Met. Survivorship curves of da-GAL4>dTsc2 and +>dTsc2 reared on ( c ) 1.0X diet containing 0.2 or 1 mM Met, ( d ) 0.4X diet containing 0.2 or 1 mM Met. 0.2 and 1 correspond to 0.2 mM Met and 1 mM Met, respectively. ( e , f ) The mean lifespan of da-GAL4>dInRDN and +>dInRDN reared on ( e ) 1.0X diet containing 0.2 or 1 mM Met (mean±s.e.m., n =81~106, *** P< 0.0001, log-rank test), ( f ) 0.4X diet containing 0.2 or 1 mM Met (mean±s.e.m., n =88~106, *** P< 0.0001, log-rank test). ( g , h ) The mean lifespan of da-GAL4>dTsc2 and +>dTsc2 reared on ( g ) 1.0X diet containing 0.2 or 1 mM Met (mean±s.e.m., n =104~149, *** P< 0.0001, log-rank test), ( h ) 0.4X diet containing 0.2 or 1 mM Met (mean±s.e.m., n =111~152, *** P< 0.0001, log-rank test). See Supplementary Tables 12 and 13 for n number and statistics of individual strains and dietary groups. ( i ) Model of TORC1 activation by Met and amino acids. Full size image As shown above, an imbalance in amino acids suppressed the lifespan extension effect of Met restriction ( Fig. 4 and Supplementary Tables 4–6 ). If Met restriction inhibits TOR signalling, the high amino-acid status may affect TOR signalling, blocking the lifespan extension by Met restriction. Surprisingly, overexpression of InRDN or Tsc2 did not extend lifespan on 0.2 mM- and 1 mM-1.0X diets ( da-Gal4 > UAS-dInRDN on the 0.2-mM Met-1.0X, −7.25%, P =0.07; da-Gal4 > UAS-dInRDN on the 1 mM Met-1.0X, −3.11%, P =0.98; da-Gal4 > UAS-dTsc2 on the 0.2 mM Met-1.0X, −7.65%, P =0.02; da-Gal4 > UAS-dTsc2 on the 1 mM Met-1.0X, −6.98%, P =0.15, log-rank test) ( Fig. 8e–h and Supplementary Tables 12 and 13 ). On the other hand, overexpression of InRDN or Tsc2 led to lifespan extension on the 1 mM Met-0.4X diet ( da-Gal4 > UAS-InRDN on the 1 mM Met-0.4X, 15.14%, P< 0.0001; da-Gal4 > UAS-Tsc2 on the 1 mM Met-0.4X, 18.65%, P< 0.0001, log-rank test), whereas no lifespan extension was observed on the 0.2 mM Met-0.4X ( da-Gal4 > UAS-dInRDN on the 0.2 mM Met-0.4X, −3.49%, P =0.07; da-Gal4 > UAS-dTsc2 on the 0.2 mM Met-0.4X, −10.90%, P< 0.0001, log-rank test) ( Fig. 8e–h and Supplementary Tables 12 and 13 ). These data indicate that delaying the aging process by inhibiting TOR signalling depends on the interaction of Met with other amino acids. Thus, the reason Met restriction was not effective in increasing lifespan under conditions of high amino acids is due to interference of the effects of Met restriction, TOR inhibition and amino-acid imbalance. It is thought that nutritional deficiency decreases fecundity and increases lifespan through redistribution of nutrient resources, and that food supplies restore egg production leading to a reduction in lifespan [28] . However, a recent study reported that the addition of Met under conditions of dietary dilution increased reproduction without affecting lifespan [21] . Our results involving fully defined diets explain this unexpected finding and relate it to both the trade-off idea and the still controversial role of Met restriction in regulating lifespan. Indeed, Met deficiency on most diets with defined and variable amino-acid status (0.7X and 1.0X) reduced reproduction, but it was not associated with lifespan extension. On the other hand, we found that Met deficiency can lead to a decrease, increase or no change in lifespan depending on the status of other dietary amino acids. Excess amino acids may lead to ineffectiveness of nutritional resource redistribution under conditions of Met restriction, whereby a decrease in reproduction may not necessarily lead to lifespan extension. Defining the mechanisms linking cost-of-reproduction to lifespan has been a long-held question in the aging field. As such, the observed diversity of responses that characterize the trade-off and involve the interplay between Met and other amino acids offers important mechanistic insights with regard to regulation of the trade-off and the aging process. By varying both total amino-acid levels and the levels of Met, we demonstrated that the lifespan extension by Met restriction requires low amino-acid status, and this finding was also held in yeast. Together with the previous data in rodents, our data suggest that Met restriction may be viewed as a general strategy to extend lifespan. The data further suggest that the lifespan regulation by Met restriction involves TOR signalling and that high levels of amino acids suppress the lifespan extension conferred by Met restriction or overexpression of InRDN or Tsc2. TORC1 (TOR complex 1) is a sensor of amino acids [29] , [30] , [31] , [32] ; therefore, it is not surprising that accumulation of amino acids activates TOR. However, a question remains regarding the mechanism of the differential inhibition of the Met effect upon changes in amino-acid status. We suggest that free amino acids may activate TOR, fully or partially, independent of Tsc1–Tsc2, while Met acts on TOR through the Tsc1–Tsc2 complex ( Fig. 8i ). Recently, the RagA/B-RagC/D GTPase complex was found to tether Rags to the lysosome in response to amino acid sensing by TORC1 and couple this signalling to proteins downstream of TORC1. This signal transduction for activation of TORC1, mediated by sensing amino acids, is independent of the Tsc1–Tsc2 complex [30] , [31] . Hence, it is possible that saturated activation of TORC1 by amino-acid accumulation may occur independently of Tsc1–Tsc2 and not be reversed by InRDN/Tsc2 overexpression or Met restriction. However, because Met is also an amino acid, it—when at low levels—may inhibit TORC1 independent of Tsc1–Tsc2. We hypothesize that the lifespan extension by Met restriction may involve other mechanisms for the following reasons: first, reduced reproduction and protein synthesis in response to Met restriction may lead to an accumulation of other amino acids, and thus free amino acids may be increased by Met restriction. This suggests that Met restriction may not use the same mechanism of amino-acid restriction for lifespan extension. Second, Met is a key regulator of reproduction and protein synthesis. Thus, Met may be involved in other regulatory functions, such as control of energy and stress. Third, TORC1 can transmit energy and stress signals sensed by the Tsc1–Tsc2 complex. Fourth, microarray data show that Met restriction-induced genes are involved in the response to toxins, lipid metabolism and steroid metabolism, all of which are relevant to regulation of energy and stress ( Fig. 6c ). Although this hypothesis needs further testing, there is increasing evidence that the mechanism of Met restriction may be independent of general amino-acid sensing by the TORC1 complex ( Fig. 8i ). Fly stocks and husbandry D. melanogaster (Canton-S, Oregon-R and w 1118 strain) lines were from the laboratory of Dr Lawrence G. Harshman (University of Nebraska, Lincoln, NE, USA). UAS-dTsc2 , UAS-dInRDN , w 1118 and da-GAL4 strains were from the laboratory of Dr Pankaj Kapahi (Buck Institute for Research on Aging, Novato, CA, USA) [9] . Flies were maintained on corn meal food, commonly used in our laboratory, and kept in a temperature-controlled chamber at 25 °C with 12-h light/dark cycle and ~60% humidity for all experiments. Newly emerged flies were transferred to fresh corn meal food and allowed to mate for 1–2 days. Virgin flies were collected at 18 °C within 16 h after eclosion and then kept on corn meal food until lifespan analyses. Three-day-old mated flies were collected using etherization, sorted by sex and then some of them were transferred to cages on the designed diet for lifespan study. Three-day-old virgin flies were also transferred to cages on the designed diet and their lifespan was analysed. Unless otherwise stated, experimental flies were held on the designed diet and transferred to fresh vials without anaesthesia every 3 days. Fly culture media In order to maintain strains and collect flies for lifespan studies, we used corn meal food (85.7 g corn meal ‘Aunt Jemina’ (The Quaker Oats Company, Chicago, IL, USA), 50 ml golden A unsulfured molasses (Groeb Farms Inc, Onsted, MI, USA), 71.4 g Torula yeast (MP Biomedicals, Solon, OH, USA), 2.86 g p-hydroxybenzoic acid methyl ester (Sigma), 6.4 g agar (MoorAgar Inc, Loomis, CA, USA) and 5.7 ml propionic acid (Sigma) per litre water). In order to test lifespan of flies, fully defined medium was used based on the fruit fly basal mix developed in a recent study [19] with modification in the amino-acid content. This diet contained 62.08 g Diet TD.04310 (corresponds to the 0.1X diet) and/or 101.07 g Diet TD.10417 (corresponds to the 1.0X diet; Harlan Teklad), 100 mg lecitin from soybean (Sigma), 500 mg ribonucleic acid from Torula yeast (Sigma), 100 g of dextrose, 20 g agar, 2.85 ml propionic acid, 0.255 ml of phosphoric acid (Sigma) and indicated amounts of Met (Sigma) per litre of water. To prepare 0.4X and 0.7X diets, the two basal mixes were mixed to adjust amino-acid concentrations. Lifespan and egg production analyses Newly hatched flies were collected within 18 h at 18 °C and kept on corn meal food at a density of 35 animals per vial. To prepare mated female flies, the flies were incubated for 24 h under the mixed sex conditions. In a typical lifespan trial, 3-day-old flies were placed in cages. The cages were made of plastic 1 l cups with grommets for changing food vials and slits for removal of dead flies by aspiration. A total of 35–70 males and/or 35–70 females were kept in each cage for testing lifespan on the fully defined medium. Three to six replica cages were used for each lifespan. Fresh food was supplied into cages and the dead flies were removed by aspiration and counted every 3 days. The control and experimental group trials were always performed concurrently. Flies were maintained in a temperature-controlled incubator at 25 °C with 12-h light/dark cycle and 50–60% humidity. Flies were also prepared for the reproduction assay following the outline of the aging experiment. Then, egg production by animals maintained on diets containing four different levels of amino acids (0.1X, 0.4X, 0.7X, 1.0X) with varying Met (0, 0.15, 1, 1.5, 10 and 100 mM) was counted, for eggs produced within 24 h, every 3 days until animals stopped laying eggs. Each vial contained five female and five male flies, and four to five replicate vials on each diet were used to count egg production. Finally, the data were represented as cumulative egg production for 30 days as well as lifetime egg production. Yeast aging replicative lifespan assays Wild-type strain BY4741 ( MAT a his3 leu2 met15 ura3 ) was used in replicative aging assays. Nitrogen-based Synthetic Defined Yeast Media (SD media) including an amino-acid mix lacking Met was used to assay lifespan under conditions of Met restriction. Met varied from 0.005 to 1 mg ml −1 , whereas all other components were kept constant. To analyse how amino-acid status affects lifespan, nitrogen-based dropout media (YNB media) and an amino-acid supplement mix without Met (CSM-Met; MP Biomedicals) were mixed before plate preparation. YNB concentration was 6.7 g l −1 and the concentration of amino-acid mix without Met varied from 0.2X to 5X. Met was added as indicated concentrations. Since our wild-type strain was an auxotroph for uracil, histidine and leucine, we also added these amino acids separately and kept them constant. For replicative aging assays, cells were grown on fresh medium overnight. For each strain, 30 daughter cells (starter mothers) were collected and assayed on agar plates. New buds (daughters) from these starter mothers were removed and discarded as they formed. This process continued until the cells stopped dividing. Lifespan was determined as the total number of daughter cells that each mother cell generated. Food consumption Mated female flies were prepared following the outline of the aging experiment and reared on diets with different amino-acid levels (0.1X, 0.4X, 0.7X, 1.0X) and varying in Met (0, 0.15, 1 and 10 mM). For the feeding assay, 0.1% (w/v) erioglaucine (FD&C Blue no. 1, Sigma) was added to each defined diet, and 6- and 21-day-old flies were fed these diets for 6 h or 30 min (12 noon–6 pm or 12 noon–12:30 pm) [33] , [34] , [35] . Five female flies per group (20 groups were used for 30-min incubation) were homogenized in 200 μl of phosphate-buffered saline, and the homogenate was centrifuged at 13,000 r.p.m. for 15 min. Absorbance of the supernatant was measured at 625 nm, with 675 nm used as a reference, and then compared with the absorbance of the control food, prepared in the same way, to calculate consumed food mass. Analysis of total protein and Met concentration Twenty-one-day-old mated female flies were prepared following the outline of the aging experiment on diets with three different levels of amino acids (0.4X, 0.7X, 1.0X) and varying Met (0, 0.15, 1, 10 mM). Twenty-five flies per group were used to determine weight. These flies were then homogenized in phosphate-buffered saline in order to measure total protein by using the BCA protein assay reagent (Pierce). To measure endogenous Met concentration in mated female flies, we followed a previously established procedure [36] , [37] . Briefly, homogenized samples were precipitated by mixing with 5% trichloroacetic acid. After incubation at 4 °C for 10 min and centrifugation at 13,000 r.p.m. for 15 min, the supernatant (50 μl) was diluted 10-fold with distilled water and prepared for OPA derivatization. The derivatization reagent was freshly prepared. Sample solutions (2–5 μl) were mixed with the OPA derivatization reagent to 100 μl final volume. Following a 2-min reaction at room temperature, 50 μl of the mixture were injected onto a Zorbax Eclipse XDB-C18 column (4.6 × 150 mm) and analysed by HPLC. Detection was by fluorescence of Met derivatives using a Waters 474 scanning fluorescence detector with excitation at 330 nm and emission at 445 nm. Fly samples for microarray analysis Newly hatched flies were collected within 18 h at 18 °C and kept on corn meal food at density of 35 animals per vial. To prepare mated female flies, collected flies were incubated for 24 h under the mixed sex conditions. Three-day-old flies were placed in vials. Twenty female flies were kept in each vial on the fully defined medium for 18 days. Ten replica vials were used for sample collection. Fresh food was supplied every 3 days and dead flies were removed by aspiration. Flies were maintained in a temperature-controlled incubator at 25 °C with 12-h light/dark cycle and 50–60% humidity. Mated female Canton-S flies raised on four different defined media were subjected to RNA extraction. Total RNA was extracted from 20 flies by Trizol (Invitrogen), according to the manufacturer’s suggestions. Extracted RNA was additionally purified by either MEGAclear of RNAqueous kit (Ambion) to ensure highest purity for microarrays. Microarray analysis was performed by using Drosophila Genome 2.0 at the microarray core of Dana-Farber Cancer Institute. Fluorescence intensity of each transcript was normalized. Expression data from Affymetrix microarrays were analysed with the dCHIP software with default settings [38] , [39] . Changes in transcript levels were compared among four sample sets of RNA. To examine changes in expression, the data were filtered with 50 permutation testing to assess False Discovery Rate as follows: (1) E/B>1.2 or B/E>1.2 and (2) E-B>100 or B-E>100 (E: Experiment, B: Baseline) or for more stringent comparison: (1) E/B>1.8 (or 1.5) or B/E>1.8 (or 1.5) and (2) E-B>100 or B-E>100 (E: Experiment, B: Baseline). Statistical analysis Statistical analyses were performed using the JMP (version 10) software (SAS Institute Inc.). Log-rank tests were used for Drosophila survival analysis. Wilcoxon rank-sum test was used for the analyses of yeast replicative lifespan. Comparisons of the means were made using Student’s t -test. How to cite this article: Lee, B. C. et al. Methionine restriction extends lifespan of Drosophila melanogaster under conditions of low amino-acid status. Nat. Commun. 5:3592 doi: 10.1038/ncomms4592 (2014).